The nuclear orphan receptor Nr4a2 induces Foxp3 and regulates differentiation of CD4+T cells Regulatory T cells (Tregs) have a central role in maintaining immune homoeostasis through various mechanisms. Although the Forkhead transcription factor Foxp3 defines the Treg cell lineage and functions, the molecular mechanisms of Foxp3 induction and maintenance remain elusive. Here we show that Foxp3 is one of the direct targets of Nr4a2. Nr4a2 binds to regulatory regions of Foxp3, where it mediates permissive histone modifications. Ectopic expression of Nr4a2 imparts Treg-like suppressive activity to naïve CD4 + T cells by inducing Foxp3 and by repressing cytokine production, including interferon-γ and interleukin-2. Deletion of Nr4a2 in T cells attenuates induction of Tregs and causes aberrant induction of Th1, leading to the exacerbation of colitis. Nr4a2-deficeint Tregs are prone to lose Foxp3 expression and have attenuated suppressive ability both in vitro and in vivo . Thus, Nr4a2 has the ability to maintain T-cell homoeostasis by regulating induction, maintenance and suppressor functions of Tregs, and by repression of aberrant Th1 induction. Regulatory T cells (Tregs), which are characterized by the expression of Foxp3, have indispensable roles in immunological tolerance, protecting the host from autoimmune diseases and allergies [1] . Foxp3 is specifically expressed in Tregs and plays a critical role in the differentiation, maintenance and effector functions of Tregs [2] . The presence of Foxp3 in Tregs is essential, as demonstrated by the fatal autoimmune disorders that occur in both humans and mice with Foxp3 gene inactivation [3] , [4] . Foxp3 is also sufficient to confer Treg-like suppressive activity on ectopic expression in non-Tregs [5] . Foxp3 is transiently induced by transforming growth factor (TGF)-β in naïve T cells, which are called induced Tregs (iTregs) [6] , whereas thymus-derived Tregs are called nTregs (natural occurring Tregs). We recently demonstrated that Smad2 and Smad3 are redundantly essential for the induction of Foxp3 in iTregs [7] . The mechanisms underlying Foxp3 expression have been extensively analysed. For Foxp3 regulation, a proximal promoter and three intronic enhancers, designated conserved noncoding sequences (CNSs) 1, 2 and 3, have been identified. The proximal promoter has potential binding sites for transcription factors including c-Rel and FoxO [8] , [9] . CNS1, which has binding sites for Smads and NF-AT, is critical for iTreg induction [10] , [11] . CNS2 contains a hypomethylated CpG island, which is essential for Foxp3 maintenance, and binding sites for Stat5, Runx/CBFβ, FoxO and c-Rel as well as Foxp3 itself [11] , [12] , [13] , [14] . CNS3 binds to c-Rel and is important for the initiation of Foxp3 expression [8] , [11] . Among the enhancer-interacting factors that have been identified, very few have been analysed in terms of their direct effect on epigenetic modification, because the ectopic expression of each factor triggers insufficient induction of Foxp3. Nr4a2 belongs to the Nr4a family of transcription factors, and exhibits a high similarity to the other two members, Nr4a1 and Nr4a3, especially in its DNA-binding domain ( ∼ 91–95% identity). Although Nr4a belongs to the nuclear receptors superfamily, their activity is not considered to be regulated by ligands, because their ligand-binding pockets are hidden by bulky amino acids, and their ligand-binding domains are constitutively active [15] . Thus, their functions are assumed to be regulated largely at the expression level, although various post-translational modifications have also been reported to modulate their functions [16] , [17] . The Nr4a family has important roles in various physiological and pathological events [18] , [19] , [20] , [21] . Several disorders are associated with the dysfunction of Nr4a, including metabolic syndromes and Parkinson's disease [18] , [19] . In this study, we demonstrated that ectopic expression of Nr4a2 in naïve CD4 + T cells along with T-cell receptor (TCR) stimulation was sufficient for the induction of Foxp3 and for the suppression of effector cytokine production, imparting Treg-like suppressive activity to naïve T cells. Through further analysis with Nr4a2-deficient animals and cells, we revealed that Nr4a2 was crucial in regulating the Th1/Treg balance, Treg lineage maintenance and effector functions of Tregs, contributing to immune homoeostasis. Ectopic expression of Nr4a2 induces Foxp3 To isolate the genes relevant to Treg induction, especially in the thymus, we first examined the 'Treg signature genes,' which were categorized into seven clusters according to their dependence on Foxp3, TGF-β, TCR stimulation and interleukin (IL)-2 for their expression [22] . We were interested in one cluster, designated 'cluster 6' by Hill et al . [22] ; the genes are enriched in Tregs, but their expression is independent of TGF-β or Foxp3 transduction. These genes are predicted to induce Foxp3. We isolated transcription factors in cluster 6 and investigated their ability to transactivate the Foxp3-luciferase reporter construct [23] ( Supplementary Fig. S1 ). Among these, Nr4a2 had the strongest potential to activate the Foxp3 promoter. We confirmed that the expression levels of Nr4a2 were higher in Foxp3 + Tregs than in Foxp3 − T cells at both the protein and mRNA levels ( Fig. 1a ). Nr4a2 was low in naïve T cells, but was transiently induced by TCR stimulation ( Fig. 1b ). Nr4a2 was undetectable in Th1, Th2, Th17 or iTreg cells differentiated in vitro ( Supplementary Fig. S2 ). 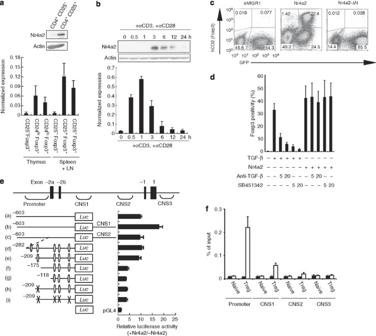Figure 1: Nr4a2 is highly expressed in Treg subsets and directly induces Foxp3. (a) Top: Nr4a2 protein expression in Tregs (CD4+CD25+) and in the Tconv (CD4+CD25–) population. Bottom: quantitative PCR (qPCR) analysis of Nr4a2 expression in CD4+T cell subsets, normalized against Hprt. (b) Naïve T cells were incubated under TCR stimulation with anti-CD3, CD28 antibodies. The protein level at each indicated time point was analysed by western blotting. Bottom: qPCR results depict the induction of Nr4a2 by TCR stimulation. Data are normalized against Hprt. (c) Effects of expression of Nr4a2 (indicated by GFP expression, which is synergistically expressed by IRES in the eMIGR1 vector) and its transactivation-deficient mutant Nr4a2-ΔN, which lacks the N terminus 237aa of the transactivation domain28, on Foxp3 expression eMIGR1, an empty vector, was used as a negative control. Foxp3 induction was detected with an anti-human CD2 (hCD2) antibody, which recognizes membranous hCD2 protein coexpressed with endogenous Foxp3 in the Foxp3-hCD2-hCD52-KI mice. Numbers in FACS plots represent percentages of CD4+T cells in the gated area. (d) Effects of blocking TGF-β signalling with a chemical inhibitor (SB431542, at 5 or 20 μM) or TGF-β neutralizing antibodies, at 5 or 20 μg ml−1on TGF-β or Nr4a2-mediated Foxp3 induction. (e) Foxp3 promoter and enhancer-driven luciferase reporter constructs were transfected into the 293 cell line. Regions with consensus binding sequences for Nr4a are indicated by open ovals. (f) ChIP assay of Nr4a2 in theFoxp3promoter and enhancer regions in naive CD4+T cells and Tregs. Cell lysates were immunoprecipitated with anti-Nr4a2 (open bars) or control IgG (filled bars). Values are presented as the percentage of corresponding input with the standard deviation (s.d.) of three independent experiments of triplicate. Numbers in FACS plots represent percentages of CD4+T cells in the gated area. Data shown in (a,b,d,e) are representative of three independent experiments (mean and s.d. of triplicate). Figure 1: Nr4a2 is highly expressed in Treg subsets and directly induces Foxp3. ( a ) Top: Nr4a2 protein expression in Tregs (CD4 + CD25 + ) and in the Tconv (CD4 + CD25 – ) population. Bottom: quantitative PCR (qPCR) analysis of Nr4a2 expression in CD4 + T cell subsets, normalized against Hprt. ( b ) Naïve T cells were incubated under TCR stimulation with anti-CD3, CD28 antibodies. The protein level at each indicated time point was analysed by western blotting. Bottom: qPCR results depict the induction of Nr4a2 by TCR stimulation. Data are normalized against Hprt. ( c ) Effects of expression of Nr4a2 (indicated by GFP expression, which is synergistically expressed by IRES in the eMIGR1 vector) and its transactivation-deficient mutant Nr4a2-ΔN, which lacks the N terminus 237aa of the transactivation domain [28] , on Foxp3 expression eMIGR1, an empty vector, was used as a negative control. Foxp3 induction was detected with an anti-human CD2 (hCD2) antibody, which recognizes membranous hCD2 protein coexpressed with endogenous Foxp3 in the Foxp3-hCD2-hCD52-KI mice. Numbers in FACS plots represent percentages of CD4 + T cells in the gated area. ( d ) Effects of blocking TGF-β signalling with a chemical inhibitor (SB431542, at 5 or 20 μM) or TGF-β neutralizing antibodies, at 5 or 20 μg ml −1 on TGF-β or Nr4a2-mediated Foxp3 induction. ( e ) Foxp3 promoter and enhancer-driven luciferase reporter constructs were transfected into the 293 cell line. Regions with consensus binding sequences for Nr4a are indicated by open ovals. ( f ) ChIP assay of Nr4a2 in the Foxp3 promoter and enhancer regions in naive CD4 + T cells and Tregs. Cell lysates were immunoprecipitated with anti-Nr4a2 (open bars) or control IgG (filled bars). Values are presented as the percentage of corresponding input with the standard deviation (s.d.) of three independent experiments of triplicate. Numbers in FACS plots represent percentages of CD4 + T cells in the gated area. Data shown in ( a , b , d , e ) are representative of three independent experiments (mean and s.d. of triplicate). Full size image Next, we investigated the ability of Nr4a2 to induce Foxp3. We ectopically expressed Nr4a2 in mouse CD4-single-positive (SP) cells by retroviral transduction and measured Foxp3 expression. Foxp3 expression was monitored using cells isolated from the knock-in mouse strain Foxp3-hCD2-hCD52-KI , in which human CD2 (hCD2) is coexpressed with Foxp3 (ref. 24 ), and can be monitored by surface staining with anti-hCD2 antibodies. Nr4a2 strongly induced Foxp3, but its transactivation-deficient mutant did not ( Fig. 1c ), despite its higher expression ( Supplementary Fig. S3 ). This Nr4a2-mediated induction of Foxp3 was independent of TGF-β in the culture media, because inhibition of TGF-β signalling with neutralizing antibodies [25] or with a chemical inhibitor of TGF-β [26] did not affect Foxp3 induction by Nr4a2, whereas these are effective in iTreg inhibition ( Fig. 1d ). We searched for the Nr4a2-responsive element of the foxp3 promoter/enhancer using a reporter assay. By constructing the deletion series of the promoter–reporters from the 5′ to 3′ direction (the 3′ border was fixed at +12), we found that the −209 to +12 promoter region was the minimal responsive region to Nr4a2 ( Fig. 1e ). As for the binding sites for Nr4a, several sequences have recently been identified [27] , in addition to the canonical binding elements [28] , [29] , [30] . We found five potential Nr4a-binding elements between −209 and +12, and identified the most important element between −209 and −175 (see e, f, h constructs in Fig. 1e and Supplementary Fig. S4 ). Insertion of CNS1 enhanced promoter activity twofold, although CNS2 did not ( Fig. 1e ). This observation was supported by ChIP analyis ( Fig. 1f ), wherein the strongest binding of Nr4a2 was to the proximal promoter, but did not to CNS3 in Tregs. Moderate binding was observed in CNS1, and weaker binding was observed in CNS2. These data indicate that Nr4a2 acts mainly on the proximal promoter and also weakly on CNS1. Nr4a2 induces epigenetic modification of histones We investigated the effect of Nr4a2 on the epigenetic status of the foxp3 promoter/enhancer. First, we isolated the total green fluorescence protein (GFP)-positive fractions from Nr4a2-virus- or control-virus-transduced CD4-SP cells, and performed native ChIP to compare their histone modification status with those of Tregs and naïve CD4 + T cells. 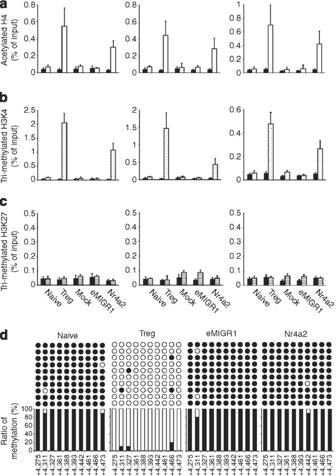Figure 2: Nr4a2 induces Treg-like active histone modifications inFoxp3regulatory regions. (a–c) Native ChIP assay ofFoxp3promoter (left), CNS1 (middle) and CNS2 (right) enhancers was performed with antibodies against modified histones (a: anti-acetylated H4, open bars;b: anti-tri-methylated H3K4, dotted bars;c: anti-tri-methylated H3K27, striped bars) and control IgG (filled bars). Naïve T cells, Tregs, mock-transduced cultured cells and sorted GFP+cells from the population of eMIGR1 or eMIGR1-Nr4a2 retrovirus-transduced cells were analysed. Values are depicted as the percentage of corresponding input. Data are representative of two independent experiments (mean and s.d. of triplicate). (d) Bisulphite sequencing revealed that Nr4a2 can not mediate the demethylation of the CpG island in the CNS2 region of thefoxp3locus. Sequencing was performed against the bisulphite-treated genomic DNA from naïve T cells, Tregs, sorted GFP+cells from the eMIGR1 retrovirus-transduced cells and sorted GFP+Foxp3+cells from the eMIGR1-Nr4a2 retrovirus-transduced cells. Ten CG sites in the CNS2 locus, located at the indicated positions, were analysed. Top: closed and open circles indicate methylated and unmethylated CG sites, respectively. Bottom: data shown in top panels were quantitated, and shown as percentages of methylation at each position. Data are pooled from two independent experiments. Foxp3+cells were sorted with APC-conjugated anti-hCD2 antibody unless otherwise indicated. As depicted in Figure 2a–c , Nr4a2 induced active histone modifications, histone H4-acetylation and histone H3K4-trimethylation, similar to the patterns in Tregs. H3K27-trimethylation, a repressive histone modification was not detected in both Tregs and Nr4a2-transduced T cells. Figure 2: Nr4a2 induces Treg-like active histone modifications in Foxp3 regulatory regions. ( a – c ) Native ChIP assay of Foxp3 promoter (left), CNS1 (middle) and CNS2 (right) enhancers was performed with antibodies against modified histones ( a : anti-acetylated H4, open bars; b : anti-tri-methylated H3K4, dotted bars; c : anti-tri-methylated H3K27, striped bars) and control IgG (filled bars). Naïve T cells, Tregs, mock-transduced cultured cells and sorted GFP + cells from the population of eMIGR1 or eMIGR1-Nr4a2 retrovirus-transduced cells were analysed. Values are depicted as the percentage of corresponding input. Data are representative of two independent experiments (mean and s.d. of triplicate). ( d ) Bisulphite sequencing revealed that Nr4a2 can not mediate the demethylation of the CpG island in the CNS2 region of the foxp3 locus. Sequencing was performed against the bisulphite-treated genomic DNA from naïve T cells, Tregs, sorted GFP + cells from the eMIGR1 retrovirus-transduced cells and sorted GFP + Foxp3 + cells from the eMIGR1-Nr4a2 retrovirus-transduced cells. Ten CG sites in the CNS2 locus, located at the indicated positions, were analysed. Top: closed and open circles indicate methylated and unmethylated CG sites, respectively. Bottom: data shown in top panels were quantitated, and shown as percentages of methylation at each position. Data are pooled from two independent experiments. Foxp3 + cells were sorted with APC-conjugated anti-hCD2 antibody unless otherwise indicated. Full size image Because the CpG island in the CNS2 is highly demethylated during Treg development, we investigated the effects of Nr4a2 on the CpG methylation status of this region. Bisulphite sequencing of Nr4a2-induced Foxp3 + cells and Tregs revealed that Nr4a2 could not induce demethylation of CNS2 ( Fig. 2d ). The results of these epigenetic experiments suggest that Nr4a2 induces Foxp3 in CD4 + T cells by mediating active histone modifications. Nr4a2 can induce Foxp3 and repress Th1 differentiation Because Nr4a mediates various physiological events, some in a redundant manner and others in a non-redundant manner, we compared the ability of the three family members to induce Foxp3. Importantly, both Nr4a1 and Nr4a3 have also been reported to be abundant in Tregs [31] and inducible by TCR stimulation [32] . We found that Nr4a1 rarely induced Foxp3, whereas Nr4a3 did so to an intermediate degree ( Fig. 3a,b ), despite the expression levels of these proteins were similar ( Supplementary Fig. S3a ). 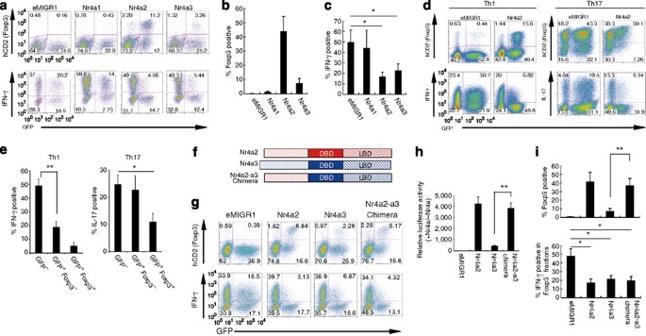Figure 3: Nr4a families vary in their ability to induce Foxp3 and to repress IFN-γ. (a) Top row: effects of Nr4a1, Nr4a2 and Nr4a3 expression on Foxp3 expression. Bottom row: effects of Nr4a1, Nr4a2 and Nr4a3 expression on IFN-γ expression. eMIGR or eMIGR-Nr4a retrovirus-transduced cells were restimulated with phorbol myristate acetate (PMA) and ionomycine at 60 h after infection for 8 h. (b,c) Quantification of the results ofa. (d) Effects of Nr4a2 transductions on Foxp3 expression (top row) and IFN-γ repression (bottom row) under Th1 and Th17 conditions. (e) Quantification of the results of the eMIGR-Nr4a2 retrovirus-transduced cells ind. (f) Schematic representation of Nr4a2, Nr4a3 and the chimeric protein of Nr4a3 in which the N-terminal of Nr4a3 is replaced with that of Nr4a2 (Nr4a2-a3 chimera). DBD, DNA-binding domain; LBD, ligand-binding domain. (g) Foxp3 induction (top row) and IFN-γ repression (bottom row) by Nr4a2, Nr4a3 and Nr4a2-a3 chimera. Cells were transduced with eMIGR1- or eMIGR1-Nr4a-retorviruses, and Foxp3 induction and IFN-γ repression were analysed. (h) Transcriptional activities as monomers of Nr4a2, Nr4a3 and Nr4a2-a3 chimera were demonstrated using NBRE-luc in 293T cells. (i) Quantification of the result ing. Numbers in FACS plots represent percentages of CD4+T cells in the gated area. Data in (b,c,e,h,i) are representative of three independent experiments (mean and s.d. of triplicate). *P< 0.05 and **P<0.01 (two-tailed Student'st-test). Figure 3: Nr4a families vary in their ability to induce Foxp3 and to repress IFN-γ. ( a ) Top row: effects of Nr4a1, Nr4a2 and Nr4a3 expression on Foxp3 expression. Bottom row: effects of Nr4a1, Nr4a2 and Nr4a3 expression on IFN-γ expression. eMIGR or eMIGR-Nr4a retrovirus-transduced cells were restimulated with phorbol myristate acetate (PMA) and ionomycine at 60 h after infection for 8 h. ( b , c ) Quantification of the results of a . ( d ) Effects of Nr4a2 transductions on Foxp3 expression (top row) and IFN-γ repression (bottom row) under Th1 and Th17 conditions. ( e ) Quantification of the results of the eMIGR-Nr4a2 retrovirus-transduced cells in d . ( f ) Schematic representation of Nr4a2, Nr4a3 and the chimeric protein of Nr4a3 in which the N-terminal of Nr4a3 is replaced with that of Nr4a2 (Nr4a2-a3 chimera). DBD, DNA-binding domain; LBD, ligand-binding domain. ( g ) Foxp3 induction (top row) and IFN-γ repression (bottom row) by Nr4a2, Nr4a3 and Nr4a2-a3 chimera. Cells were transduced with eMIGR1- or eMIGR1-Nr4a-retorviruses, and Foxp3 induction and IFN-γ repression were analysed. ( h ) Transcriptional activities as monomers of Nr4a2, Nr4a3 and Nr4a2-a3 chimera were demonstrated using NBRE-luc in 293T cells. ( i ) Quantification of the result in g . Numbers in FACS plots represent percentages of CD4 + T cells in the gated area. Data in ( b , c , e , h , i ) are representative of three independent experiments (mean and s.d. of triplicate). * P < 0.05 and ** P <0.01 (two-tailed Student's t -test). Full size image In microglia, Nr4a2 has been shown to repress inflammatory cytokines [33] . Therefore, we analysed the effects of Nr4a on the production of the Th1-effector cytokine interferon (IFN)-γ. Interestingly, Nr4a2 and Nr4a3, which induced Foxp3, also strongly repressed IFN-γ ( Fig. 3a,c ). Nr4a1, in contrast, could not repress IFN-γ. In microglia, Nr4a2 repressed cytokines in a DNA-binding-independent manner [33] . However, the C280A/E281A mutant, which lacks the DNA-binding activity [33] , could no longer induce Foxp3 or repress IFN-γ ( Supplementary Fig. S3b ), suggesting that Nr4a2 must bind DNA directly, to execute both functions. We further analysed Foxp3 and cytokine regulation by Nr4a2 under Th1- and Th17-conditions. Both IFN-γ and IL-17 were significantly repressed under Th1- and Th17-conditions, respectively, and Foxp3 was induced in both conditions by Nr4a2 ( Fig. 3d ). Importantly, the Nr4a2-mediated repression of IFN-γ occurred even in Foxp3-negative fractions, and the induced Foxp3 further repressed IFN-γ ( Fig. 3e ). In contrast, IL-17 repression was detected only in the Foxp3-positive fraction ( Fig. 3e ). These results indicate that Nr4a2 has the ability to repress Th1 differentiation by both Foxp3-independent and -dependent mechanisms. We further investigated the differences between the Nr4a proteins at the molecular level through domain swapping analysis. When the amino (N) terminus of Nr4a3 was replaced with that of Nr4a2 ( Fig. 3f ), the resulting chimeric construct affected transcriptional activity at a level equivalent to that of Nr4a2 ( Fig. 3h ). Importantly, the chimeric construct also exhibited a similar level of Foxp3 induction ( Fig. 3g,i ), indicating that the intrinsic transcriptional activity in the N terminus distinguishes Nr4a2 and Nr4a3. Similar domain swapping also imparted significant Foxp3 induction and IFN-γ repression ability to Nr4a1 ( Supplementary Fig. S3c ). However, the effects were not as strong as those of Nr4a2, indicating functions in carboxy terminus also distinguish Nr4a1 and Nr4a2. Nr4a2-induced Foxp3 + cells have in vitro suppression activity Next, we characterized Nr4a2-induced Foxp3 + cells by analysing the expression profile of Treg effectors and suppression activity. Expression levels of Foxp3 mRNA in Nr4a2-induced Foxp3 + cells were one-quarter to one-third of that in restimulated Tregs ( Fig. 4a ). IL-2 was completely repressed, and CD25 , a subunit of the high affinity Il-2 receptor complex, was higher than that in Tregs, suggesting that Nr4a2-induced Foxp3 + cells can consume IL-2 by ligand–receptor interactions, similar to Tregs. Although TGF-β1 and GITR were highly expressed in the Nr4a2-induced Foxp3 + cells, IL-10 was repressed, and CTLA-4 required a long interval for induction. These data indicate that Nr4a2-induced Foxp3 + cells expressed similar but distinctive set of Treg effectors. 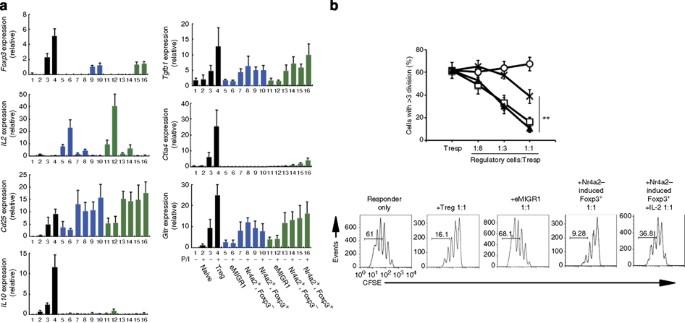Figure 4: Nr4a2 induces suppression activityin vitroby upregulating CD25 and repressing IL-2. (a) qPCR analysis of the effects of Nr4a2 expression on the expression of Treg effector genes. mRNA was prepared from naïve T cells (columns 1 and 2), Tregs (columns 3 and 4), the GFP+fraction of eMIGR1 retrovirus-transduced cells (columns 5, 6, 11 and 12), and the GFP+Foxp3–(columns 7, 8, 13 and 14) or GFP+Foxp3+(columns 9, 10, 15 and 16) fraction of eMIGR1-Nr4a2 retrovirus-transduced cells, which were incubated with (even-numbered columns) or without (odd-numbered columns) PMA/ionomycine for 2 h. Retrovirus-transduced cells were sampled at 48 h (blue bars, columns 5 to 10) and 84 h (green bars, columns 11 to 16) after infection. Expression levels of the indicated mRNA, are presented relative to theHprtexpression. Data are representative of three independent experiments (mean and s.d. of triplicate). (b)In vitrosuppression assay. Top: suppression of CFSE-labeled naïve CD4+T cells (responder, Tresp) by Tregs (open squares), the GFP+fraction of eMIGR1 retrovirus-transduced cells (open circles), the GFP+Foxp3+fraction of eMIGR1-Nr4a2 retrovirus-transduced cells (filled triangles), or the GFP+Foxp3+fraction of eMIGR1-Nr4a2 retrovirus-transduced cells supplemented with IL-2 (5 ng ml−1, crosses). Cells were cultured for 96 h with anti-CD3/anti-CD28-coated beads. The ratio of responder cells with more than three divisions are presented. Bottom: results in the top panel at the 1:1 ratio of regulatory cells/Tresp are presented. Numbers in FACS plots represent percentages of CD4+T cells in the gated area. Data are representative of three independent experiments (mean and s.d. of triplicate). **P<0.01 (two-tailed Student′st-test). Figure 4: Nr4a2 induces suppression activity in vitro by upregulating CD25 and repressing IL-2. ( a ) qPCR analysis of the effects of Nr4a2 expression on the expression of Treg effector genes. mRNA was prepared from naïve T cells (columns 1 and 2), Tregs (columns 3 and 4), the GFP + fraction of eMIGR1 retrovirus-transduced cells (columns 5, 6, 11 and 12), and the GFP + Foxp3 – (columns 7, 8, 13 and 14) or GFP + Foxp3 + (columns 9, 10, 15 and 16) fraction of eMIGR1-Nr4a2 retrovirus-transduced cells, which were incubated with (even-numbered columns) or without (odd-numbered columns) PMA/ionomycine for 2 h. Retrovirus-transduced cells were sampled at 48 h (blue bars, columns 5 to 10) and 84 h (green bars, columns 11 to 16) after infection. Expression levels of the indicated mRNA, are presented relative to the Hprt expression. Data are representative of three independent experiments (mean and s.d. of triplicate). ( b ) In vitro suppression assay. Top: suppression of CFSE-labeled naïve CD4 + T cells (responder, Tresp) by Tregs (open squares), the GFP + fraction of eMIGR1 retrovirus-transduced cells (open circles), the GFP + Foxp3 + fraction of eMIGR1-Nr4a2 retrovirus-transduced cells (filled triangles), or the GFP + Foxp3 + fraction of eMIGR1-Nr4a2 retrovirus-transduced cells supplemented with IL-2 (5 ng ml −1 , crosses). Cells were cultured for 96 h with anti-CD3/anti-CD28-coated beads. The ratio of responder cells with more than three divisions are presented. Bottom: results in the top panel at the 1:1 ratio of regulatory cells/Tresp are presented. Numbers in FACS plots represent percentages of CD4 + T cells in the gated area. Data are representative of three independent experiments (mean and s.d. of triplicate). ** P <0.01 (two-tailed Student′s t -test). Full size image Next, we performed an in vitro suppression assay to functionally characterize the Nr4a2-induced Foxp3 + cells. The Nr4a2-induced Foxp3 + cells in this assay efficiently suppressed the proliferation of TCR-stimulated naïve CD4 + T cells ( Fig. 4b ). This strong in vitro suppression activity was mainly mediated by the IL-2 consumption, which has been suggested to be a central mechanism for in vitro suppression by Tregs [34] , because supply of IL-2 in the medium significantly attenuated the suppression ( Fig. 4b ). Nr4a2 induces iTregs and represses aberrant Th1 induction The findings above suggest the involvement of Nr4a2 in Foxp3 induction and Th1 suppression. To analyse the roles of Nr4a2 in T-cell development and differentiation, we crossed Nr4a2-floxed mice with Lck-Cre + mice, which express Cre-recombinase specifically in T cells [35] , [36] . Although more than half of the Nr4a2 fl/fl Lck-Cre + mice died neonatally with unknown reasons, surviving mice developed normally and were fertile, and had no symptoms of autoimmune diseases up to 4 months of age. However, the population of CD44highCD62Llow-activated CD4 + T cells, as well as that of IFN-γ + cells were significantly increased in Nr4a2 fl/fl Lck-Cre + mice compared with Nr4a2 +/+ Lck-Cre + littermates. On the other hand, the number of Tregs in the thymus and spleen was not altered in the Nr4a2 fl/fl Lck-Cre + mice ( Supplementary Fig. S5a,b ). We isolated naïve CD4 + T cells from Nr4a2 fl/fl Lck-Cre + and Nr4a2 +/+ Lck-Cre + mice, and cultured them under neutral, Th1-, Th17- and iTreg-skewing conditions. We observed strong induction of Th1 under all culture conditions, and a decrease in iTreg and Th17 induction ( Fig. 5a ). Expression levels of Foxp3 protein were also lower in Nr4a2-deficient iTreg cells ( Fig. 5b ). These results are consistent with forced expression studies, which indicate the involvement of Nr4a2 in Th1 repression and Foxp3 induction. 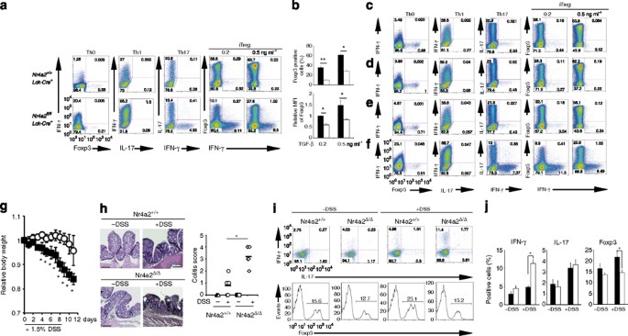Figure 5: Deletion of Nr4a2 attenuates iTreg induction. (a) Effects of Nr4a2-knockout on CD4+T cells differentiation. iTreg induction was carried out at the two different TGF-β concentrations indicated. Naïve CD4+T cells fromNr4a2+/+Lck-Cre+orNr4a2fl/flLck-Cre+mice were cultured under the indicated conditions for 96 h. IFN-γ, Foxp3 or IL-17 expressions were analysed. (b) Quantification of the results inaof the iTreg condition at 0.2 and 0.5 ng ml−1TGF-β. Top: ratio of the Foxp3+fractions. Bottom: mean fluorescence intensity (MFI) of Foxp3-staining of the Foxp3+fractions. The value ofNr4a2+/+Lck-Cre+cells at 0.2 ng ml−1TGF-β was set to 1. Data are representative of three independent experiments (mean±s.d. in triplicate). Filled bars:Nr4a2+/+Lck-Cre+cells; open bars:Nr4a2fl/flLck-Cre+cells. (c–f) Effects of theex vivodeletion of Nr4a2 on Th and iTreg differentiation. Isolated naïve CD4+T cells fromNr4a2+/+ERT2-Cre+(c,d) orNr4a2fl/flERT2-Cre+(e,f) mice were treated (d,f) or untreated (c,e) with 4-hydroxy tamoxifen for 6 h in RPMI1640 10% FBS at 37 °C. Cells were cultured under the indicated conditions for 96 h. IFN-γ, Foxp3 or Il-17a expression were analysed. (g) Body weight ofNr4a2+/+Lck-Cre+(open circles) orNr4a2fl/flLck-Cre+(filled squares) mice treated with 1.5% DSS. Data are representative of two independent experiments, each with five mice per group (mean±s.d. of five mice). (h) Histological analysis of the experiments of (g) at day 11. Top: hematoxylin and eosin staining of colon sections. Scale bar, 100 μm. Bottom: histological score of colitis. Data are representative of two independent experiments, each with five mice per group (vertical bars: median of the colitis scores). (i) Analysis of colon and caecum lamina proprial CD4+T cells from the experiments ingat day 11, examining IFN-γ and IL-17a expression (top) and Foxp3 expression (bottom). (j) Quantification of results ini. Data are representative of two independent experiments, each with five mice per group (mean±s.d. of five mice). Filled bars:Nr4a2+/+Lck-Cre+mice; open bars:Nr4a2fl/flLck-Cre+mice. Numbers in FACS plots represent percentages of CD4+T cells in the gated area. *P<0.05, **P<0.01 (two-tailed Student'st-test). Figure 5: Deletion of Nr4a2 attenuates iTreg induction. ( a ) Effects of Nr4a2-knockout on CD4 + T cells differentiation. iTreg induction was carried out at the two different TGF-β concentrations indicated. Naïve CD4 + T cells from Nr4a2 +/+ Lck-Cre + or Nr4a2 fl/fl Lck-Cre + mice were cultured under the indicated conditions for 96 h. IFN-γ, Foxp3 or IL-17 expressions were analysed. ( b ) Quantification of the results in a of the iTreg condition at 0.2 and 0.5 ng ml −1 TGF-β. Top: ratio of the Foxp3 + fractions. Bottom: mean fluorescence intensity (MFI) of Foxp3-staining of the Foxp3 + fractions. The value of Nr4a2 +/+ Lck-Cre + cells at 0.2 ng ml −1 TGF-β was set to 1. Data are representative of three independent experiments (mean±s.d. in triplicate). Filled bars: Nr4a2 +/+ Lck-Cre + cells; open bars: Nr4a2 fl/fl Lck-Cre + cells. ( c – f ) Effects of the ex vivo deletion of Nr4a2 on Th and iTreg differentiation. Isolated naïve CD4 + T cells from Nr4a2 +/+ ERT2-Cre + ( c , d ) or Nr4a2 fl/fl ERT2-Cre + ( e , f ) mice were treated ( d , f ) or untreated ( c , e ) with 4-hydroxy tamoxifen for 6 h in RPMI1640 10% FBS at 37 °C. Cells were cultured under the indicated conditions for 96 h. IFN-γ, Foxp3 or Il-17a expression were analysed. ( g ) Body weight of Nr4a2 +/+ Lck-Cre + (open circles) or Nr4a2 fl/fl Lck-Cre + (filled squares) mice treated with 1.5% DSS. Data are representative of two independent experiments, each with five mice per group (mean±s.d. of five mice). ( h ) Histological analysis of the experiments of ( g ) at day 11. Top: hematoxylin and eosin staining of colon sections. Scale bar, 100 μm. Bottom: histological score of colitis. Data are representative of two independent experiments, each with five mice per group (vertical bars: median of the colitis scores). ( i ) Analysis of colon and caecum lamina proprial CD4 + T cells from the experiments in g at day 11, examining IFN-γ and IL-17a expression (top) and Foxp3 expression (bottom). ( j ) Quantification of results in i . Data are representative of two independent experiments, each with five mice per group (mean±s.d. of five mice). Filled bars: Nr4a2 +/+ Lck-Cre + mice; open bars: Nr4a2 fl/fl Lck-Cre + mice. Numbers in FACS plots represent percentages of CD4 + T cells in the gated area. * P <0.05, ** P <0.01 (two-tailed Student's t -test). Full size image As Nr4a2 is deleted early in T-cell development in the thymus of Nr4a2 fl/fl Lck-Cre + mice, these differences in CD4 + T-cell differentiation may merely reflect the altered nature of naïve T cells. To exclude this possibility, we used naïve CD4 + T cells from Nr4a2 fl/fl ERT2-Cre + mice, in which the Nr4a2 alleles can be deleted ex vivo with tamoxifen (4-hydroxy tamoxifen) treatment. We confirmed the appropriate deletion of Nr4a2 with 6 h treatment with 4-hydroxy tamoxifen in vitro, specifically in Nr4a2 fl/fl ERT2-Cre + CD4 + T cells ( Supplementary Fig. S5c ). The results of the in vitro differentiation experiments were similar to those obtained with Lck-Cre ( Fig. 5c–f ), confirming that Nr4a2 in naïve T cells is necessary for iTreg induction and suppression of aberrant induction of Th1. To evaluate the importance of the Nr4a2-mediated regulation of CD4 + T-cell differentiation at pathological conditions in vivo, we analysed a mouse model of inflammatory bowel disease in Nr4a2 fl/fl Lck-Cre + mice. Dextran sulphate sodium (DSS)-treatment significantly accelerated body weight loss and induced severe intestinal inflammation in Nr4a2 fl/fl Lck-Cre + compared with Nr4a2 +/+ Lck-Cre + mice ( Fig. 5g,h ). Furthermore, we observed a significant increase in the number of Th1 cells and the attenuated increase of Treg population in colon and caecum lamina propria in Nr4a2 fl/fl Lck-Cre + mice treated with DSS ( Fig. 5i,j ). These data indicate that Nr4a2 is important for Treg induction and suppression of aberrant Th1 induction, also at pathological conditions in vivo . Nr4a2 is critical for sustained expression of Foxp3 Next, we analysed the roles of Nr4a2 in Tregs by breeding Nr4a2-floxed mice with Foxp3 YFP-Cre mice [36] , [37] to knockout Nr4a2 specifically in Tregs. We confirmed the specific deletion of Nr4a2 in Tregs ( Supplementary Fig. S6a ). Nr4a2 fl/fl Foxp3 YFP-Cre mice were apparently normal, disease free and without differences in the activation status of CD4 + T cells ( Supplementary Fig. S6b ). In the first experiment, we compared the relative sizes of Nr4a2-sufficient and Nr4a2-deficient Tregs population in Nr4a2 +/+ Foxp3 YFP-Cre/+ , heterozygous Nr4a2 fl/+ Foxp3 YFP-Cre/+ and homozygous Nr4a2 fl/fl Foxp3 YFP-Cre/+ females ( foxp3 is on X chromosome). The YFP + /YFP – ratio in Nr4a2 +/+ Foxp3 YFP-Cre/+ mice was near 1:1 in both thymus and periphery ( Fig. 6a,b ). However, in Nr4a2 fl/fl Foxp3 YFP-Cre/+ mice, ratios of YFP + /YFP − were suboptimal ( ∼ 0.3 in thymus and ∼ 0.1 in periphery, Fig. 6a,b ), indicating that Tregs were not properly maintained on deletion of Nr4a2 . The YFP + /YFP − ratio in Nr4a2 fl/+ Foxp3 YFP-Cre/+ mice was near ∼ 0.8 in thymus, and ∼ 0.4 in periphery, indicating that Tregs are not properly maintained even by the heterozygous deletion of Nr4a2 ( Fig. 6b ). Importantly, the ratio of YFP + /YFP − in Nr4a2 fl/fl Foxp3 YFP-Cre/+ mice decreased with age ( Supplementary Fig. S6c ), supporting the idea that the disequilibrium is caused by the accelerated reduction of the Nr4a2-deficient Tregs in the periphery, rather than the reduced positive selection of Tregs in the thymus. Another possibility which could explain this disequilibrium might be reduced export of Nr4a2-deficient Tregs, although we think it less probable, because the reduced export is expected to result in an increase in the number of Nr4a2-deficient Tregs in the thymus. Deletion of Nr4a1 did not affect the YFP + /YFP − ratio in Tregs ( Fig. 6a,b and Supplementary Fig. S6d ), indicating that Nr4a1 does not contribute to Treg homoeostasis; this corresponds well with the observation that Nr4a1-transduction did not induce Foxp3 ( Fig. 3a ). The CpG methylation status of CNS2, an important determinant of Treg lineage stability, was not perturbed in Nr4a2 fl/fl Lck-Cre + mice ( Supplementary Fig. S6e ), suggesting that Nr4a2 is not essential for the demethylation of CNS2 during nTreg development. This was consistent with our forced expression study ( Fig. 2d ). 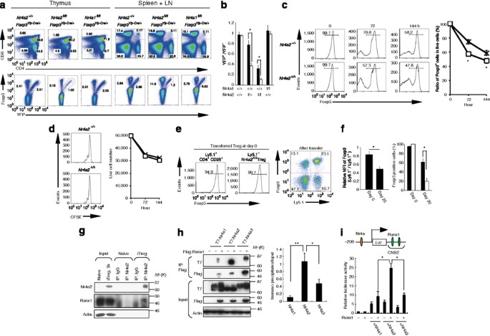Figure 6: Nr4a2 stabilizes Foxp3 expression in Tregs. (a) Top: CD4+and CD8+compartments of whole cells from the indicated organs. Bottom: Foxp3 and YFP expression in CD4-SP fractions in top. (b) Quantification of the results ina. Ratio of YFP+/YFP–in total Foxp3+cells. Filled bars: results of thymus; open bars: results of spleen plus lymph nodes. Data are pooled from three independent experiments, with six mice from each genotype total, aged 11- to 13 weeks (mean±s.d.). (c) Left: CFSE-labeled CD4+CD25+YFP+Tregs fromNr4a2+/+Foxp3Yfp-Cre/+orNr4a2fl/flFoxp3Yfp-Cre/+mice, cultured under neutral condition with 20 ng ml−1IL-2, thymidine (2 mM) and z-VAD-fmk (10 μM) were analysed for Foxp3 expression at the time indicated. YFP-fluorescences were bleached by fixation/permeabilization. Right: quantification of the results in left. Open squares:Nr4a2fl/flFoxp3Yfp-Crecells; crosses:Nr4a2+/+Foxp3Yfp-Crecells. (d) Proliferation and survival status of cells inc. Left: CFSE dilution of live cells at 144 h. Right: live cell number at indicated time points. Open squares:Nr4a2fl/flFoxp3Yfp-Crecells; crosses:Nr4a2+/+Foxp3Yfp-Crecells. (e) Rag2–mice were co-transferred with 3×105CD4+CD25+YFP+Ly5.2+Tregs fromNr4a2fl/flFoxp3Yfp-Cremice and 3×105CD4+CD25+Ly5.1+wild-type Tregs. Foxp3 expression at day 0 and days 20 after transfer are shown. (f) Quantification of the results ine. Left: mean fluorescence intensity (MFI) of Foxp3-staining of the Foxp3+fractions. Right: ratio of Foxp3-positive fractions. Closed bars: cells in Ly5.1+fractions; open bars: cells in Ly5.1−fractions. Data are pooled from two independent experiments with five mice from each sample set total (mean±s.d.). (g) Coimmunoprecipitation of Nr4a2 and Runx1 from total cell lysates of naïve CD4+T cells, or of naïve CD4+T cells stimulated under the iTreg condition. (h) Left: coimmunoprecipitation of Flag-Runx1 and T7-Nr4a in 293T cell lysates. Right: quantification of the result in left. Intensity of the anti-T7 blot of the anti-Flag immunoprecipitates, normalized with the anti-T7 input. (i) Top: schematic representation of the reporter construct. Nr4a-binding site and the Runx1-binding sites are indicated. Bottom: results of the luciferase assay. Numbers in FACS plots represent percentages of cells in the gated area. Data are representative of three (c,h,i) or two (d) independent experiments (mean±s.d. of triplicate). *P< 0.05, **P<0.01 (two-tailed Student'st-test). Figure 6: Nr4a2 stabilizes Foxp3 expression in Tregs. ( a ) Top: CD4 + and CD8 + compartments of whole cells from the indicated organs. Bottom: Foxp3 and YFP expression in CD4-SP fractions in top. ( b ) Quantification of the results in a . Ratio of YFP + /YFP – in total Foxp3 + cells. Filled bars: results of thymus; open bars: results of spleen plus lymph nodes. Data are pooled from three independent experiments, with six mice from each genotype total, aged 11- to 13 weeks (mean±s.d.). ( c ) Left: CFSE-labeled CD4 + CD25 + YFP + Tregs from Nr4a2 +/+ Foxp3 Yfp-Cre/+ or Nr4a2 fl/fl Foxp3 Yfp-Cre/+ mice, cultured under neutral condition with 20 ng ml −1 IL-2, thymidine (2 mM) and z-VAD-fmk (10 μM) were analysed for Foxp3 expression at the time indicated. YFP-fluorescences were bleached by fixation/permeabilization. Right: quantification of the results in left. Open squares: Nr4a2 fl/fl Foxp3 Yfp-Cre cells; crosses: Nr4a2 +/+ Foxp3 Yfp-Cre cells. ( d ) Proliferation and survival status of cells in c . Left: CFSE dilution of live cells at 144 h. Right: live cell number at indicated time points. Open squares: Nr4a2 fl/fl Foxp3 Yfp-Cre cells; crosses: Nr4a2 +/+ Foxp3 Yfp-Cre cells. ( e ) Rag2 – mice were co-transferred with 3×10 5 CD4 + CD25 + YFP + Ly5.2 + Tregs from Nr4a2 fl/fl Foxp3 Yfp-Cre mice and 3×10 5 CD4 + CD25 + Ly5.1 + wild-type Tregs. Foxp3 expression at day 0 and days 20 after transfer are shown. ( f ) Quantification of the results in e . Left: mean fluorescence intensity (MFI) of Foxp3-staining of the Foxp3 + fractions. Right: ratio of Foxp3-positive fractions. Closed bars: cells in Ly5.1 + fractions; open bars: cells in Ly5.1 − fractions. Data are pooled from two independent experiments with five mice from each sample set total (mean±s.d.). ( g ) Coimmunoprecipitation of Nr4a2 and Runx1 from total cell lysates of naïve CD4 + T cells, or of naïve CD4 + T cells stimulated under the iTreg condition. ( h ) Left: coimmunoprecipitation of Flag-Runx1 and T7-Nr4a in 293T cell lysates. Right: quantification of the result in left. Intensity of the anti-T7 blot of the anti-Flag immunoprecipitates, normalized with the anti-T7 input. ( i ) Top: schematic representation of the reporter construct. Nr4a-binding site and the Runx1-binding sites are indicated. Bottom: results of the luciferase assay. Numbers in FACS plots represent percentages of cells in the gated area. Data are representative of three ( c , h , i ) or two ( d ) independent experiments (mean±s.d. of triplicate). * P < 0.05, ** P <0.01 (two-tailed Student's t -test). Full size image The suboptimal YFP + /YFP − ratio in Nr4a2-floxed Foxp3 YFP-Cre/+ mice may be caused by the accelerated loss of Foxp3 expression, or by accelerated cell death or reduced proliferation. To examine these possibilities, we isolated CD4 + CD25 + YFP + Tregs from spleens and lymph nodes of Nr4a2 fl/fl Foxp3 YFP-Cre and Nr4a2 +/+ Foxp3 YFP-Cre mice, cultured them in vitro and then monitored the Foxp3 expression. To exclude the contribution of cell death and expansion of Foxp3-negative cells, we cultured the cells in the presence of thymidine and z-VAD-fmk to inhibit cell proliferation and apoptosis, respectively. We observed that the Nr4a2-deficient Tregs lost Foxp3 expression with a significantly accelerated rate compared with Nr4a2-sufficient Tregs ( Fig. 6c ). As cell proliferation and death were properly inhibited under this culture condition ( Fig. 6d ), the majority of Foxp3-negative cells that appeared after culture were direct descendants of the Foxp3 + Tregs. In addition, the Foxp3 positive fraction at 72 h of culture did not appear as sharp peaks, but as broader peaks with left 'shoulders', suggesting the presence of Treg populations with ongoing loss of Foxp3. To further investigate the role of Nr4a2 in the maintenance of Foxp3 in Tregs, we co-transferred wild-type Ly5.1 + CD4 + CD25 + Tregs ( ∼ 95% Foxp3 + ) and Nr4a2 -deficeint Ly5.2 + CD4 + CD25 + YFP + Tregs ( ∼ 99.7% Foxp3 + ) at 1:1 ratio into lymphopenic recipients. As previously reported, substantial fraction of Tregs became Foxp3-negative after homoeostatic expansion [24] . After transfer, ∼ 40% of the wild-type Ly5.1 + Tregs became Foxp3-negative, whereas almost 80% of Ly5.1 − fraction became Foxp3-negative ( Fig. 6e, f ). Importantly, although the level of Foxp3 protein expression was initially equivalent, the Nr4a2-deficient Tregs exhibited a significantly lower level of Foxp3 than wild-type Tregs after transfer ( Fig. 6f ), strongly indicating the accelerated loss of Foxp3 in the Nr4a2-deficient Tregs. Altogether, these results strongly suggest that Nr4a2 is directly involved in the Treg lineage maintenance by sustaining Foxp3 expression. Nr4a2 cooperates with Runx/Cbfβ The observed roles of Nr4a2 in Foxp3 expression is reminiscent of that of Runx/CBFβ in Treg maintenance [12] , [38] . Through coimmunoprecipitation experiments on total cell lysates from primary CD4 + T cells, we detected Runx1 in the anti-Nr4a2 immunoprecipitates, under Nr4a2-inducing conditions ( Fig. 6g ). Considering the different capacities of the three Nr4a proteins for Foxp3 induction and Treg maintenance, we compared the Nr4a's binding affinity to Runx1. T7-tagged Nr4a and Flag-tagged Runx1 were ectopically expressed in 293T cells and the lysates were immunoprecipitated with anti-Flag antibodies. Nr4a2 showed the strongest affinity to Runx1 ( Fig. 6h ). We further investigated the functional interaction between Nr4a and Runx1 by reporter assay. We used a construct composed of the Foxp3 proximal promoter, which contains the Nr4a-responsive element identified in Fig. 1e , and CNS2, which reportedly contains Runx-responsive elements [12] ( Fig. 6i ). Although Runx1 itself could not activate this reporter, it enhanced Nr4a-mediated transactivation of the reporter ( Fig. 6i ). Importantly, the strongest synergistic effect occurred when Runx1 interacted with Nr4a2. The result of the ChIP analysis in Figure 1f , which showed weak enrichment of the CNS2 in the anti-Nr4a2 immunoprecipitates from Treg, further indicated the interaction between Nr4a2 on the promoter and Runx1 on CNS2 in Tregs. Overall, these results suggest that Nr4a2 and Runx/CBFβ cooperates to maintain Treg lineage stability. Nr4a2-deficient Tregs have attenuated suppressive activity To further investigate the roles of Nr4a2 in Tregs we measured expression levels of Treg markers, activation status, cell death and proliferation in YFP + Foxp3 + and YFP – Foxp3 + Tregs in Nr4a2 +/+ Foxp3 YFP-Cre/+ and Nr4a2 fl/fl Foxp3 YFP-Cre/+ mice, which allowed us to compare Nr4a2-deficient and Nr4a2-suficient Tregs in the same mice. We observed decreased levels of Foxp3 and CD25 in YFP + fraction in Nr4a2 fl/fl Foxp3 YFP-Cre/+ mice ( Fig. 7a ). Other Treg markers such as CTLA-4 and GITR were expressed at a similar level between Nr4a2-deficient and Nr4a2-sufficient Tregs ( Fig. 7a ). A similar expression pattern of CD62L indicated equivalent activation status. A similar percentage of cells staining positive for Annexin V and Ki67 indicated an equivalent rate of cell proliferation and death between the Nr4a2-deficient and Nr4a2-sufficient Tregs, further supporting the notion that the insufficiency of the Nr4a2-deficient Tregs observed in Figure 6a,b was not caused by a difference in cell death or proliferation. We also compared the expression levels of Treg-relevant mRNA between Tregs from Nr4a2 +/+ Foxp3 YFP-Cre and Nr4a2 fl/fl Foxp3 YFP-Cre mice. We found decreased expression of Foxp3 , indicating that the accelerated loss of Foxp3 in Nr4a2-deficient Tregs was at the mRNA level ( Fig. 7b ). For other genes, we observed a significant reduction of CD25 , TGF-β1 and CCR9 . 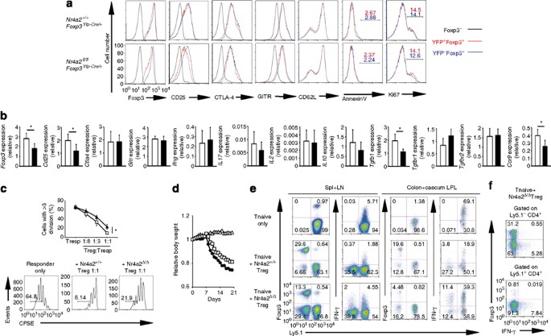Figure 7: Attenuatedin vitroandin vivosuppressive activity of Nr4a2-deficient Tregs. (a) FACS analysis of the indicated protein levels in YFP+Foxp3+and YFP–Foxp3+Tregs ofNr4a2+/+Foxp3Yfp-Cre/+orNr4a2fl/flFoxp3Yfp-Cre/+mice. For Foxp3, CD25, CTLA-4 and GITR expression levels in non-Treg cells are represented by black lines, as a negative value. Data are representative of three independent experiments (means of duplicate are shown for the positive fractions of Annexin V and Ki67 staining). (b) Comparison of mRNA levels between Tregs inNr4a2+/+Foxp3Yfp-CreandNr4a2fl/flFoxp3Yfp-Cremice. Expression levels of the indicated mRNA, are presented relative toHprtexpression. Open bars:Nr4a2+/+Foxp3Yfp-CreTregs; closed bars:Nr4a2fl/flFoxp3Yfp-CreTregs. (c) Top:in vitrosuppression assay with CFSE-labeled wild-type CD4+CD25–cells as responders and CD4+CD25+YFP+Tregs fromNr4a2+/+Foxp3Yfp-Cre(open squares) orNr4a2fl/flFoxp3Yfp-Cre(closed triangles) mice as suppressors. Ratios of responder cells with more than three divisions are presented. Bottom: results in the top panel at 1:1 Treg/Tresp ratio. (d) Body weight ofRag2–mice injected with 5×105naïve Ly5.1+CD4+T cells alone or in combination with 3×105CD4+CD25+YFP+Ly5.2+Tregs fromNr4a2+/+Foxp3Yfp-CreorNr4a2fl/flFoxp3Yfp-Cremice. Data are pooled from two independent experiments, with seven mice from each sample set total. The ranges of body weights (relative body weights to day 0) of each group at day 21 are Tnaive only: 0.69–0.76; Tnaive+Nr4a2+/+Foxp3Yfp-CreTregs: 0.96–1.08; Tnaive+Nr4a2fl/flFoxp3Yfp-CreTregs: 0.76–0.88. (e) Expression of Foxp3 and IFN-γ in CD4+T cells from the spleen and lymph nodes (left panels), and from the colon and caecum lamina propria (right panels) inRag2–recipients presented indat day 21. (f) Frequencies of IFN-γ-expressing cells in Foxp3–CD4+T cells and Foxp3+CD4+T cells from the spleen and lymph nodes ofRag2–recipients presented indat day 21. Numbers in FACS plots represent percentages of CD4+T cells in the gated area. Data inb,care representative of three independent experiments (mean and s.d. of triplicate). *P<0.05 (two-tailed Student'st-test). Figure 7: Attenuated in vitro and in vivo suppressive activity of Nr4a2-deficient Tregs. ( a ) FACS analysis of the indicated protein levels in YFP + Foxp3 + and YFP – Foxp3 + Tregs of Nr4a2 +/+ Foxp3 Yfp-Cre/+ or Nr4a2 fl/fl Foxp3 Yfp-Cre/+ mice. For Foxp3, CD25, CTLA-4 and GITR expression levels in non-Treg cells are represented by black lines, as a negative value. Data are representative of three independent experiments (means of duplicate are shown for the positive fractions of Annexin V and Ki67 staining). ( b ) Comparison of mRNA levels between Tregs in Nr4a2 +/+ Foxp3 Yfp-Cre and Nr4a2 fl/fl Foxp3 Yfp-Cre mice. Expression levels of the indicated mRNA, are presented relative to Hprt expression. Open bars: Nr4a2 +/+ Foxp3 Yfp-Cre Tregs; closed bars: Nr4a2 fl/fl Foxp3 Yfp-Cre Tregs. ( c ) Top: in vitro suppression assay with CFSE-labeled wild-type CD4 + CD25 – cells as responders and CD4 + CD25 + YFP + Tregs from Nr4a2 +/+ Foxp3 Yfp-Cre (open squares) or Nr4a2 fl/fl Foxp3 Yfp-Cre (closed triangles) mice as suppressors. Ratios of responder cells with more than three divisions are presented. Bottom: results in the top panel at 1:1 Treg/Tresp ratio. ( d ) Body weight of Rag2 – mice injected with 5×10 5 naïve Ly5.1 + CD4 + T cells alone or in combination with 3×10 5 CD4 + CD25 + YFP + Ly5.2 + Tregs from Nr4a2 +/+ Foxp3 Yfp-Cre or Nr4a2 fl/fl Foxp3 Yfp-Cre mice. Data are pooled from two independent experiments, with seven mice from each sample set total. The ranges of body weights (relative body weights to day 0) of each group at day 21 are Tnaive only: 0.69–0.76; Tnaive+ Nr4a2 +/+ Foxp3 Yfp-Cre Tregs: 0.96–1.08; Tnaive+ Nr4a2 fl/fl Foxp3 Yfp-Cre Tregs: 0.76–0.88. ( e ) Expression of Foxp3 and IFN-γ in CD4 + T cells from the spleen and lymph nodes (left panels), and from the colon and caecum lamina propria (right panels) in Rag2 – recipients presented in d at day 21. ( f ) Frequencies of IFN-γ-expressing cells in Foxp3 – CD4 + T cells and Foxp3 + CD4 + T cells from the spleen and lymph nodes of Rag2 – recipients presented in d at day 21. Numbers in FACS plots represent percentages of CD4 + T cells in the gated area. Data in b , c are representative of three independent experiments (mean and s.d. of triplicate). * P <0.05 (two-tailed Student's t -test). Full size image Then we measured suppressive activity of Nr4a2-deficeint Tregs in vitro . Tregs from Nr4a2 fl/fl Foxp3 YFP-Cre mice exhibited slightly, but significantly less suppressive activity compared with those from Nr4a2 +/+ Foxp3 YFP-Cre mice ( Fig. 7c ), possibly caused by the lower expression of CD25 (refs 34 , 39 ) and by the accelerated loss of Foxp3. Finally, to assess the suppressive activity of the Nr4a2-deficient Tregs in vivo , we analysed the transfer model of colitis. We transferred wild-type naïve Ly5.1 + CD4 + T cells alone or in combination with Ly5.2 + CD4 + CD25 + YFP + Tregs ( ∼ 99.7% purity) from Nr4a2 +/+ Foxp3 YFP-Cre or Nr4a2 fl/fl Foxp3 YFP-Cre mice, into Rag2 -deficeint recipient. Within 10 days, body weight loss and severe intestinal inflammation were found in recipients of naïve T cells, and this was prevented by Nr4a2-sufficient Treg ( Fig. 7d and Supplementary Fig. S6f ). In contrast, Nr4a2-deficient Tregs exhibited a significantly attenuated ability to inhibit the wasting disease and colitis ( Fig. 7d and Supplementary Fig. S6f ). We analysed the fate of transferred naïve T cells and Tregs according to Ly5.1 expression. We found a significant reduction in the Foxp3 + population in Ly5.1 − CD4 + fraction in the Nr4a2 -deficeint Treg-transferred recipients, whereas majority of the Nr4a2-sufficient Tregs still retain Foxp3 expression ( Fig. 7e ). In recipients with Nr4a2- deficeint Tregs, lamina proprial CD4 + T cells contained fewer Ly5.1 − cells, possibly caused by the lower expression of CCR9, a gut-tropic factor of lymphocytes [40] ( Fig. 7b,e ). In the Ly5.1 − CD4 + fraction of the Nr4a2 -deficeint Treg-transferred recipients, significant population of CD4 + T cells expressed IFN-γ ( Fig. 7e ). These IFN-γ-positive CD4 + were mainly Foxp3-negative, but some of the Foxp3-positive fraction was also IFN-γ + ( Fig. 7f ). These data indicate that Nr4a2 is essential for both lineage maintenance and full-suppression activity of Tregs. We have demonstrated the strong ability of Nr4a2 to induce Foxp3 and repress inflammatory cytokines, including IFN-γ thus regulating the Th1/Treg balance. Nr4a2 also has a role in mature Tregs by maintaining lineage stability and regulating effector molecules, including CD25 and TGF-β1. These roles are critical for maintaining immune homoeostasis, as evidenced by the exacerbation of the model diseases as a result of Nr4a2 insufficiency. To the best of our knowledge, no previously reported factor induced Foxp3 as effectively as Nr4a2 expect for TGF-β. Given this ability for Foxp3 induction, and the induction of Nr4a2 by TCR stimulation, we speculate that Nr4a2 has a role in nTreg development in the thymus. However, even in Nr4a2 fl/fl Lck-Cre + mice in which the Nr4a2 alleles were deleted during early T-cell development before the Foxp3 induction, we observed the unperturbed development of nTreg. Although this result can be simply interpreted that Nr4a2 is not essential for nTreg induction, we suggest another possibility that, Nr4a3, which also exhibits Foxp3-inducing ability, redundantly acts to induce nTreg. In contrast, we observed a significant reduction in the number of Nr4a2-deficeint nTregs compared with Nr4a2-suffceint nTregs in the same mice ( Fig. 6a ). This discrepancy might be explained by compensatory homoeostatic expansion of Tregs in Nr4a2 fl/fl Lck-Cre + mice. In contrast to the nTreg development, we observed significantly attenuated iTreg induction in vitro , with the aberrant induction of Th1. The exacerbation of colitis in DSS-treated Nr4a2 fl/fl Lck-Cre + mice provides evidence for the importance of Th1/iTreg regulation by Nr4a2. In the regulation of Th1/iTreg differentiation, Nr4a2 directly induced Foxp3 by activating the Foxp3 promoter/enhancer. Although the mechanisms of IFN-γ repression by Nr4a2 are currently undiscovered, the Foxp3 induction and the IFN-γ repression might not be separable roles of Nr4a2, because Nr4a1, which could not induce Foxp3, also could not repress IFN-γ. Nr4a2 is expected to regulate expression of several genes in CD4 + T cells. However, Foxp3 is an important target, demonstrated by the production of Foxp3 + Treg-like suppressive cells by ectopic expression of Nr4a2, and by the significant attenuation of iTreg induction and the impaired maintenance and function of Tregs by its deletion. Future studies comprehensively analysing the target genes of Nr4a2 during Treg induction should facilitate our understanding if the molecular mechanisms of Th/iTreg regulation governed by Nr4a2. The clarification of the mechanisms underlying Treg lineage maintenance is particularly important, considering the recent active debate on Treg lineage stability. It was recently reported that Tregs are mainly composed of a stable population [41] . Our study suggests that the high level of Nr4a2 contributes to the lineage stability. The importance of Nr4a2 in terms of Treg maintenance can be further speculated from our observation that Nr4a2 was not expressed in the in vitro -induced iTreg, which is an unstable cell population [42] , [43] . Although the trials to develop stable iTregs, aimed at the treatment of autoimmune diseases, allergies and successful organ transplantation seem to focus on the demethylation of CNS2 (refs 34 , 44 , 45 ), maintaining a sufficient level of Nr4a2 should also contribute to iTreg stability. Runx/CBFβ is necessary for maintaining Treg functions [12] , [38] . In this study, we observed the physical and functional interaction between Runx1 and Nr4a2. Although Runx1 alone directly upregulates IFN-γ, it represses the gene in the presence of Foxp3 (ref. 46 ). This result corresponds well with our observations that Nr4a2 represses IFN-γ and that this repression was further strengthened by Foxp3 expression. It is possible that Nr4a2 forms a ternary complex with Runx1 and Foxp3, thereby stabilizing Tregs. This phenomenon also supports the hypothesis that Foxp3 and IFN-γ are not totally separable targets of Nr4a2, but instead components of an auto-regulatory system driven by Nr4a2 and Foxp3, leading to tight repression of IFN-γ, which effectively sustains Tregs cell lineage. In addition to Runx/CBFβ, Nr4a2 may work with other foxp3 -regulators (Smads, c-Rel, Stat5 and so on), for Foxp3 induction in CD4 + T cells, because the ectopic expressions of Nr4a2 in other cell types induce distinct subsets of genes, which apparently do not contain Foxp3 (refs 18 , 47 ). We observed significant attenuation of the suppressive activity of Nr4a2-deficient Tregs in the transfer model of colitis in Rag2 –/– mice. However, the Nr4a2 fl/fl Foxp3 YFP-Cre mice did not show any inflammatory or autoimmune diseases. In the Nr4a2 fl/fl Foxp3 YFP-Cre mice, we speculate that Tregs in the lymphoid organs and intestine were maintained in normal number by homoeostatic maintenance under the specific pathogen-free condition. However, the abnormalities of the Nr4a2-deficient Tregs might be highlighted in the transfer model of colitis, an acute inflammatory disorder condition, with accelerated loss of Foxp3 during homoeostatic expansion in lymphopenic mice [24] , [40] , and the suboptimal homing of Nr4a2-deficeint Tregs to intestine after intravenous injection, due to the lower CCR9 levels. From the in vitro and in vivo suppression assays, it is indicated that Nr4a2 is also involved in the suppressive functions of Tregs by regulating effector expression. CD25 and TGF-β1 might be directly regulated by Nr4a2, because the ectopic expression of Nr4a2 upregulated both molecules, and the deletion of Nr4a2 resulted in their reduction. In conclusion, we propose that Nr4a2 be added to the list of Treg regulators, on account of the strong induction of Foxp3 and the suppressive activity by ectopic Nr4a2 in CD4 + T cells, the aberrant Th1/Treg differentiation of Nr4a2-deficient CD4 + T cells and the perturbed lineage maintenance of Nr4a2-deficient Tregs. The ability of Nr4a2 to induce Foxp3 even under Th1 or Th17 conditions, together with its ability to impart suppressive activity to CD4 + T cells, make it a potential therapeutic target for inflammatory diseases. Mice All work performed using mice was carried out in accordance with the guidelines for animal care approved by Keio University. Animals were maintained in specific pathogen-free conditions. Foxp3-hCD2-hCD52-KI mice [24] were originally from the laboratory of Dr S Hori. The Nr4a1-floxed and Nr4a2-floxed mice from Dr H Ichinose have been described elsewhere [36] . Foxp3 YFP-Cre knock-in mice were provided by Dr A Rudensky [37] . All mouse studies have been performed regardless of their sex, except for those for the epigenetic analysis of foxp3 locus, in which male mice were used. We did not obtain different results between males and females in our studies. Antibodies The monoclonal antibody against Nr4a1 (H1648) and Nr4a2 (N1404) was purchased from Perseus Proteomics. Antibodies to actin (A2066) and Flag-tag (M2) were purchased from Sigma. Anti-T7-tag polyclonal antibody (PM022) was purchased from MBL. Phycocerythrin-, PerCP-Cy5.5-, allophycocyanin (APC)- and APC-Cy7-conjugated monoclonal antibodies for CD4 (L3T4), CD8 (53-6.7), hCD2 (LFA-2), Foxp3 (FJK-16s), IFN-γ (KMG1.2), IL-2 (JES6-5H4), IL-10 (JES5-16E3) and IL-17a (eBio17B7) antibodies were purchased from eBiosciences. Anti-Runx1 antibody was purchased from Active Motif. PerCP-Cy5.5-conjugated anti-mouse Ki67 goat polyclonal antibody (M-19) was purchased from Santa Cruz. Annexin V staining was performed with Annexin V-Biotin Apoptosis Detection Kit (BioVision). Isolation of naïve T cells and Tregs For thymic CD4-SP, CD25 – T-cell preparation, thymocytes from 6- to 8-week-old mice were depleted of non-CD4-SP T cells by the application of biotin-conjugated antibodies against CD8a, B220, CD25, CD11b, CD49b, TER-119 and hCD2, at concentrations of 1 μg per 10 7 cells in combination with streptavidin microbeads, using large depletion columns (Miltenyi). CD4-SP cells were further purified with anti-CD4 magnetic beads using medium separation columns (Miltenyi). The purity of CD4-SP CD25 − Foxp3 − T cells was consistently greater than 95%. For naïve CD4 + T-cell (CD4 + CD25 – CD62L hi ) preparation from the spleen and lymph nodes, spleen and lymph node cells from 6- to 8-week-old mice were depleted of non-CD4 + T cells by the application of biotin-conjugated antibodies against CD8a, B220, CD25, CD11b, CD49b, TER-119 and hCD2, at concentrations of 1 μg per 10 7 cells in combination with streptavidin microbeads, using large depletion columns (Miltenyi). Then, cells were incubated with biotin-conjugated antibodies against CD62L, followed by incubation with streptavidin microbeads, and the CD62 hi cells were positively selected using large selection columns (Miltenyi). For Treg preparation, the spleen and lymph node cells were labelled with anti-CD4, anti-CD25 and anti-hCD2 (when using the Foxp3-hCD2-hCD52-KI mice) at a concentration of 0.5 μg ml −1 or YFP-fluorescence (when using the Foxp3 YFP-Cre mice) and triple-positive cells were sorted using a FACSAria. Culture of primary T cells Cells were cultured under neutral conditions (plate-coated anti-CD3e (2C11, 2 μg ml −1 ) and anti-CD28 (57.31, 0.5 μg ml −1 ) antibodies, IL-2 (PeproTech, 5 ng ml −1 ), 2-Mercaptoethanol (Invitrogen, 55 μM), and 10% fetal bovine serum in RPMI1640 unless otherwise indicated. For Th-skewing conditions, cells were cultured in RPMI1640 medium supplemented with plate-coated anti-CD3e (2C11, 2 μg ml −1 ), anti-CD28 (57.31, 0.5 μg ml −1 ), 2-Mercaptoethanol (Invitrogen, 55 μM) and 10% fetal bovine serum, supplemented with the following: for iTreg: anti-IFN-γ (R4-6A2, 1 μg ml −1 ), anti-IL-4 (1 μg ml −1 )) antibodies, 5 ng ml −1 IL-2 and recombinant human TGF-β (2 ng ml −1 , R&D Systems); for Th1: anti-IL-4 (1 μg ml −1 ), 5 ng ml −1 IL-2, IL-12 (PeproTech, 10 ng ml −1 ); for Th2: anti-IFN-γ (R4-6A2, 1 μg ml −1 ), 5 ng ml −1 IL-2, IL-4 (PeproTech, 10 ng ml −1 ); and for Th17: anti-IFN-γ (1 μg ml −1 ), anti-IL-4 (1 μg ml −1 ) antibodies, human IL-6 (R&D Systems, 10 ng ml −1 ), and recombinant human TGF-β1 (1 ng ml −1 R&D Systems). Protein analysis For immunoprecipitation, cells were lysed in lysis buffer (140 mM NaCl, 1% Triton X-100, 1 mM EDTA, 10 mM Tris (pH 8.0), supplemented with protease inhibitor cocktail (Nacalai Tesque)) for 1 h at 4 °C. Cell lysates were incubated with 1 μg of the appropriate antibodies for 4 h at 4 °C, then incubated with 15 μl protein G-Sepharose (GE Healthcare). Immunoprecipitates were washed five times with wash buffer (140 mM NaCl, 0.1% Triton X-100, 1 mM EDTA, 10 mM Tris (pH 8.0)). Proteins were dissolved in SDS–polyacrylamide gel electrophoresis sample buffer, then separated by SDS–polyacrylamide gel electrophoresis and electrotransferred to an Immobilon-P PDVF membrane (Millipore). Membranes were hybridized with the indicated antibodies at a concentration of 1 μg ml −1 , then visualized using an ECL-Plus detection system (GE Healthcare). mRNA preparation and quantitative PCR Total RNA was extracted using an RNeasy Micro Kit (Macherey Nagel) and subjected to reverse transcription using a High Capacity cDNA Synthesis Kit (Applied Biosystems). PCR analysis was performed with an iCycler iQ multicolor real-time PCR detection system (Bio-Rad) and a KAPA SYBR FAST qPCR Kit (Kapa Biosystems). All primer sets yielded a single product of the correct size. Relative expression levels were normalized against Hprt. Crosslinked chromatin immunoprecipitation Crosslinked chromatin immunoprecipitation were performed as follows; total cells from spleens and lymph nodes from three male mice were stained with phycocerythrin-conjugated anti-CD25 and PerCP-conjugated anti-CD4 antibodies before fixation, at 1 μg ml −1 . Cells were then fixed with 10 ml of 1% formaldehyde for 15 min with occasional swirling. Crosslinking was stopped by adding glycine to 125 mM. Cells were washed three times in PBS and dissolved in FACS buffer; afterward, CD4 + CD25 − and CD4 + CD25 + populations from male mice were sorted using a FACSAria cell sorter. Collected cells were lysed in 200 μl of a solution consisting of 20 mM Tris (pH 7.5), 5 mM EDTA and 0.5% SDS, supplemented with a protease inhibitor cocktail for 10 min while rotating at 4 °C. Genomic fragments were sonicated to a mean size of ∼ 400 bp. After insoluble material was removed through centrifugation, 50 μl of the supernatants was used as input, and the remainder was diluted fivefold in 1% Triton X-100, 2 mM EDTA, 150 mM NaCl and 20 mM Tris (pH 8.0) with a protease inhibitor cocktail. Immunoprecipitation was induced with 1 μg of anti-Nr4a2mAb or control mouse IgG overnight at 4 °C. Complexes were recovered by incubation with 20 μl of protein A agarose/Salmon Sperm DNA (Millipore) for 2 h at 4 °C. Precipitates were washed serially with 1 ml of RIPA buffer (50 mM Tris (pH 8.0), 150 mM NaCl, 0.1% SDS, 0.5% Na-deoxycholate, 1% NP-40, 1 mM EDTA), 1 ml of 50 mM Tris (pH 8.0), 500 mM NaCl, 0.1% SDS, 0.5% Na-deoxycholate, 1% NP-40, 1 mM EDTA, 1 ml of 50 mM Tris (pH 8.0), 1 mM EDTA, 250 mM LiCl, 1% NP-40 and 0.5% Na-deoxycholate, and then twice with 1 ml of TE. Chromatin samples were removed from the beads twice with 100 μl of 1% SDS and 0.1 M NaHCO 3 for 30 min at room temperature with constant agitation. After centrifugation, supernatants were treated with 0.2 mg ml −1 RNaseA for 30 min at room temperature, then with 0.2 mg ml −1 proteinase K for 5 h at 56 °C. Crosslinking was reversed by overnight incubation at 65 °C. After phenol–chloroform extraction, the aqueous phase was ethanol-precipitated and dissolved with 100 μl of TE buffer. Products were analysed by quantitative PCR. The PCR primer sets used are listed below. Isolation of lamina propria leucocytes Colons with caecums were excised and laced in ice-cold PBS. After washing out the luminal contents with PBS, colons and caecums were longitudinally opened, minced into ∼ 0.5 cm pieces and incubated in Ca- and Mg-free Hank's buffered salt solution containing 2% fetal bovine serum (FBS) and 1 mM EDTA for 45 min at 37 °C with constant agitation, to release intestinal epithelial cells. The remaining tissues were further minced into ∼ 1 mm pieces, and were digested with 0.5 mg ml −1 Collagenase D (Roche) and 0.3 mg ml −1 DNaseI in RPMI1640 10% FBS, for 1 h at 37 °C with constant agitation. Lamina propria lymphocytes (LPLs) were purified on a 37%/75% Percoll (GE Healthcare) gradient by centrifugation for 20 min at 25 °C at 600 g with no break. Transfer model of colitis Naïve CD4 + T cells (CD4 + CD25 – CD62L hi ; 5×10 5 ) alone or in combination with 3×10 5 Treg (CD4 + CD25 + YFP + Ly5.2 + ) cells from Nr4a2 +/+ Foxp3 Yfp-Cre or Nr4a2 fl/fl Foxp3 Yfp-Cre mice were intravenously injected into Rag2 –/– recipient mice. Transferred mice were monitored daily for weight loss. At day 21 post-transfer, animals were sacrificed for analysis. DSS-induced colitis Mice were given 1.5% DSS (mw 36,000–50,000; MP Biomedicals) dissolved in drinking water for 8 days, followed by the provision of normal drinking water for 3 days. Mice were monitored daily for weight loss. Bisulphite sequencing Genomic DNA extracted from ∼ 2×10 5 cells from male mice were digested with Bam HI. H 2 O was added to the 500 ng of the digested DNA to a volume of 19 μl, and 1.2 μl of 6 N NaOH was then added; the mixture was then incubated at 37 °C for 15 min. Next, 120 μl of 3.6 N sodium bisulphite, 0.57 mM hydroquinone and 0.3 N NaOH were added. Samples were then treated with 15 cycles of 95 °C for 30 s to 50 °C for 15 min. The reaction was then desalted using the Wizard DNA Clean-up System (Promega), and eluted with 50 μl of TE. Three microliters of 5 N NaOH were added and the samples were incubated for 5 min at room temperature. The products were then ethanol-precipitated and dissolved with 50 μl of TE buffer. The CNS2 region was PCR amplified with the primer set shown in supplemental materials and methods, and T/A cloned into pGEM-T Easy Vector (Promega). Ten inserted plasmids from each condition were purified and sequenced. In vitro suppression assay Responder cells (CD4 + CD25 – CD62L high ; 2×10 4 ) were labelled with 5 μM carboxyfluorescein diacetate succinimidyl diester (CFSE, Invitrogen), then cultured together with unlabelled cells at the indicated ratio for 96 h at 37 °C in 200 μl of RPMI medium plus 10% FBS, supplemented with 55 μM β-mercaptoethanol, in the presence of Dynabeads Mouse T-activator CD3/CD28 (Veritas) in round-bottomed 96-well dishes at a concentration of 1 bead per cell. CFSE dilution was analysed by flow cytometry, after quenching GFP fluorescence by fixation and permeabilization with a Foxp3 Staining Kit (eBioscience), if necessary. How to cite this article: Sekiya, T. et al . The nuclear orphan receptor Nr4a2 induces Foxp3 and regulates differentiation of CD4 + T cells. Nat. Commun. 2:269 doi: 10.1038/ncomms1272 (2011).